Pharyngeal sense organs drive robust sugar consumption inDrosophila The fly pharyngeal sense organs lie at the transition between external and internal nutrient-sensing mechanisms. Here we investigate the function of pharyngeal sweet gustatory receptor neurons, demonstrating that they express a subset of the nine previously identified sweet receptors and respond to stimulation with a panel of sweet compounds. We show that pox-neuro ( poxn ) mutants lacking taste function in the legs and labial palps have intact pharyngeal sweet taste, which is both necessary and sufficient to drive preferred consumption of sweet compounds by prolonging ingestion. Moreover, flies putatively lacking all sweet taste show little preference for nutritive or non-nutritive sugars in a short-term feeding assay. Together, our data demonstrate that pharyngeal sense organs play an important role in directing sustained consumption of sweet compounds, and suggest that post-ingestive sugar sensing does not effectively drive food choice in a simple short-term feeding paradigm. Sweet taste plays a key role in promoting ingestion of nutritionally rich sources of carbohydrates. Adult Drosophila express sweet taste receptors in gustatory receptor neurons (GRNs) located in the legs, labellum and a set of three pharyngeal sense organs collectively referred to as the internal mouthparts [1] . Sweet GRNs in the legs and labellum are broadly tuned to sugar stimuli, and their activation initiates feeding behaviours including the proboscis extension reflex (PER) [2] , [3] , [4] , [5] , [6] , [7] . However, neither the physiology nor the behavioural roles of pharyngeal GRNs have been described. The pharyngeal sense organs consist of the dorsal and ventral cibarial sense organs (DCSOs and VCSOs) and the more distal labral sense organ (LSO) [1] , [8] . The DCSO has two gustatory sensilla on each side of the midline, each housing three GRNs. Each side of the VCSO and LSO has three gustatory sensilla housing a total of eight and ten GRNs, respectively [8] , [9] . Axons from pharyngeal GRNs project via the pharyngeal nerve to the subesophageal zone (SEZ) of the brain, where they target an area that is distinct from the projections of the leg and labellar GRNs [1] , [3] . Mapping of body parts to different areas of the SEZ raises the possibility that taste detection by the legs, labellum and pharyngeal sense organs may each have distinct ethological functions. The Drosophila genome encodes 68 members of the gustatory receptor (Gr) family, with nine classified as sweet receptors [2] , [3] , [4] , [5] , [6] , [7] , [10] , [11] , [12] , [13] . Eight of these, Gr5a, Gr61a and Gr64a–64f, are closely related in sequence and are the defining members of a clade of insect sweet taste receptors [14] . Both expression and functional analyses suggest that sweet GRNs co-express multiple sweet receptors [4] , [10] , [11] , [13] , [15] . Furthermore, mapping of Gr promoter-GAL4 expression patterns to identified sensilla in the labellum and tarsi suggests that individual sweet Grs may be expressed in overlapping but distinct subsets of sweet GRNs [8] , [9] , [16] , [17] . In addition to the sweet clade, a highly conserved receptor, Gr43a, also functions as a sugar receptor [5] , [13] , [18] . Interestingly, Gr43a, which is expressed in a few neurons in the protocerebrum, appears to be restricted to some tarsal and pharyngeal GRNs in the gustatory system [13] , [16] , [17] . In addition to sweet taste, mounting evidence suggests that the caloric content of sugars can drive feeding preferences in both insects and mammals [19] , [20] , [21] , [22] , [23] , [24] , [25] , [26] . To distinguish between the nutritional and gustatory effects of various sugars, it would be beneficial to examine animals that completely lack taste sensory input [19] , [21] , [22] . One proposed means of achieving this effect in flies has been to use pox-neuro ( poxn ) mutants, in which external taste bristles are transformed into mechanosensory bristles [21] , [22] , [27] , [28] . However, there is evidence that the pharyngeal sense organs of poxn mutants retain expression of at least some gustatory genes [29] . If poxn mutants have functional pharyngeal taste sensilla, this could account for their observed preference for caloric sugars [21] , [22] . Here we attempt to parse out the distinctions between external and internal sugar sensing by examining the role of pharyngeal taste in the fly. We show that the pharyngeal sense organs include several GRNs that express sweet taste receptors and respond to sweet compounds. We also demonstrate that poxn mutants have functional pharyngeal sweet GRNs, and use silencing of these neurons in the poxn mutant background to examine the effects of taste and nutrient sensing on feeding decisions. We find that flies lacking all identified sweet GRN function lose most of their preference for sweet compounds in a simple short-term binary choice assay. Our results suggest that taste is the primary influence on short-term feeding decisions and that post-ingestive sugar sensing plays at most only a minor role in this context. Pharyngeal GRNs express sweet receptors Previous studies have suggested that sweet receptors are expressed in internal pharyngeal GRNs [4] , [13] , [30] . To assign selected sweet receptors to identified pharyngeal GRNs, we used seven previously reported Gr promoter-GAL4 transgenes [16] , [17] and a LexA knock-in allele of Gr64f [13] . Mapping was based on the examination of green fluorescent protein (GFP) expression in the LSO, VCSO and DCSO of flies carrying each Gr-GAL4 or Gr LexA driver, as well as analysis of GFP expression in flies carrying two different drivers. Six of the seven sweet Gr-GAL4 drivers, as well as Gr64f LexA , showed expression in the pharynx and suggest that the LSO and VCSO are innervated by sweet GRNs ( Fig. 1 ). We did not detect any Gr5a-GAL4 expression in the pharynx, and none of the sweet Gr-GAL4 lines tested showed expression in the DCSO (not shown). The map identifies two candidate sweet GRNs per side of the LSO, which co-express Gr43a and Gr64e with other members of the sweet clade. The VCSO also contains two candidate sweet GRNs per side, both of which express Gr43a-GAL4 and Gr64e-GAL4 . Thus, Gr43a-GAL4 and Gr64e-GAL4 offer two tools to explore the physiological and behavioural roles of the pharyngeal sense organs. Both are expressed in all identified candidate pharyngeal sweet neurons, as well as GRNs in the legs; however, Gr64e-GAL4 is also expressed in the taste hairs and taste pegs of the labellum, while Gr43a-GAL4 lacks labellar expression, but is expressed in sugar-sensing neurons in the protocerebrum [13] , [16] , [17] , [30] . 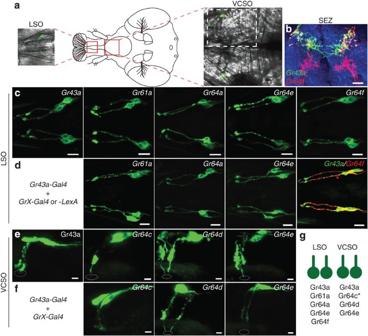Figure 1: Pharyngeal GRNs express sweet Grs. (a) Diagram showing the positions of the LSO and VCSO, with associated images of each structure from a fly expressing GFP under control ofGr43a-GAL4. Dotted white box indicates area shown ine–f. (b) Axonal projections ofGr43a-GAL4(green) andGr64fLexA(red) to the SEZ. Overlapping regions are from LSO projections. (c)Gr-GAL4-driven GFP expression in LSO. Scale bars, 10 μm (c,d). (d) LSO GFP expression from flies carryingGr43a-GAL4and indicated secondGr-GAL4orGr64fLexA. (e)Gr-GAL4-driven GFP expression in VCSO. (f) VCSO GFP expression from flies carryingGr43a-GAL4and indicated second Gr-GAL4. Scale bars, 5 μm ine–f. Dotted circles indicate the cuticular pore of sensilla. (g) Schematic of observed sweet Gr expression in LSO and VCSO GRNs. Asterisk indicates thatGr64c-GAL4expression is seen in only one neuron per side of the VCSO. Figure 1: Pharyngeal GRNs express sweet Grs. ( a ) Diagram showing the positions of the LSO and VCSO, with associated images of each structure from a fly expressing GFP under control of Gr43a-GAL4 . Dotted white box indicates area shown in e – f . ( b ) Axonal projections of Gr43a-GAL4 (green) and Gr64f LexA (red) to the SEZ. Overlapping regions are from LSO projections. ( c ) Gr-GAL4 -driven GFP expression in LSO. Scale bars, 10 μm ( c , d ). ( d ) LSO GFP expression from flies carrying Gr43a-GAL4 and indicated second Gr-GAL4 or Gr64f LexA . ( e ) Gr-GAL4 -driven GFP expression in VCSO. ( f ) VCSO GFP expression from flies carrying Gr43a-GAL4 and indicated second Gr-GAL4. Scale bars, 5 μm in e – f . Dotted circles indicate the cuticular pore of sensilla. ( g ) Schematic of observed sweet Gr expression in LSO and VCSO GRNs. Asterisk indicates that Gr64c-GAL4 expression is seen in only one neuron per side of the VCSO. Full size image Pharyngeal GRNs detect a variety of sugars To examine the role of sweet taste detected by the pharyngeal sense organs, we began by measuring the response properties of pharyngeal neurons expressing Gr43a. We expressed GCaMP3 under the control of Gr43a-GAL4 and used an in vivo imaging preparation to measure the calcium responses of GRN axon terminals in the SEZ during consumption of sweet stimuli ( Fig. 2 ). Pharyngeal Gr43a + GRNs exhibited broad tuning to sweet compounds, with responses to both nutritive (sucrose, fructose and glucose) and non-nutritive (arabinose and L -fucose) sugars, as well as the sweet sugar alcohol glycerol ( Fig. 2e ). Consistent with the reported lack of Gr5a expression in the pharyngeal sense organs, we did not observe responses to the Gr5a ligand trehalose [3] , [4] , [5] . We also saw no response to the nutritive sugar alcohol sorbitol, which is generally considered tasteless to the fly. Taken together, these data confirm that, as predicted by their Gr expression, a subset of pharyngeal GRNs is activated by the ingestion of sweet compounds. In addition, it is notable that calcium responses in pharyngeal GRNs were sustained much longer than those previously observed from stimulation of labellar GRNs [6] , [31] . 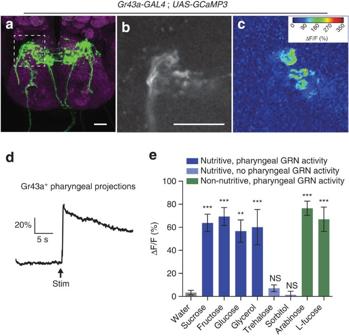Figure 2: Pharyngeal GRNs respond to sweet compounds. (a) Immunofluorescence of anti-GFP (green) and nc82 (magenta) in the SEZ of flies expressing GCaMP3 under control ofGr43a-GAL4. Dotted line shows area imaged inb. (b) Single-optical section of baseline GCaMP3 fluorescence in pharyngeal GRN axon terminals. Scale bars, 20 μm (a,b). (c) Heat map showing change in GCaMP3 fluorescence during ingestion of 1 M fructose. (d) Representative trace of fluorescence change of GCaMP3 in Gr43a axon terminals during ingestion of 1 M fructose. Arrow indicates time at which stimulus is applied to the proboscis to initiate feeding. (e) Peak fluorescence changes of GCaMP3 in Gr43a axon terminals during ingestion of 1 M solutions of the indicated compounds. Values represent mean±s.e.m. forn=5 flies per stimulus (n=4 for sorbitol), with data collected over at least 2 days. Asterisks indicate significant difference from water by one-way analysis of variance with Bonferroni correction for multiple comparisons: **P<0.01, ***P<0.001; NS, not significant. Figure 2: Pharyngeal GRNs respond to sweet compounds. ( a ) Immunofluorescence of anti-GFP (green) and nc82 (magenta) in the SEZ of flies expressing GCaMP3 under control of Gr43a-GAL4 . Dotted line shows area imaged in b . ( b ) Single-optical section of baseline GCaMP3 fluorescence in pharyngeal GRN axon terminals. Scale bars, 20 μm ( a , b ). ( c ) Heat map showing change in GCaMP3 fluorescence during ingestion of 1 M fructose. ( d ) Representative trace of fluorescence change of GCaMP3 in Gr43a axon terminals during ingestion of 1 M fructose. Arrow indicates time at which stimulus is applied to the proboscis to initiate feeding. ( e ) Peak fluorescence changes of GCaMP3 in Gr43a axon terminals during ingestion of 1 M solutions of the indicated compounds. Values represent mean±s.e.m. for n =5 flies per stimulus ( n =4 for sorbitol), with data collected over at least 2 days. Asterisks indicate significant difference from water by one-way analysis of variance with Bonferroni correction for multiple comparisons: ** P <0.01, *** P <0.001; NS, not significant. Full size image poxn mutants retain functional pharyngeal sense organs To investigate the behavioural role of internal pharyngeal GRNs, we began by examining null mutants for the transcription factor poxn . poxn mutants lack external taste bristles, which are instead transformed into mechanosensory bristles [28] . This has resulted in the use of poxn mutants as taste-blind flies [21] , [22] . However, the pharyngeal sense organs of poxn mutants have been reported to express a reporter for the apparently gustatory-specific odorant-binding protein, OBP56b , raising the possibility that taste sensilla may be intact in these tissues [29] . Moreover, many of the neurons in the pharyngeal organs of the adult originate in the embryo and persist through the larval stages and metamorphosis, which contrasts with the general principle that adult sensory structures are born during metamorphosis and suggests that the pharyngeal organs may depend on an entirely distinct developmental program [9] . We, therefore, began by asking whether poxn mutants have functional pharyngeal taste sensilla. Transheterozygotes for two poxn null alleles ( poxn 70 and poxn ΔM22-B5 ) showed normal expression of Gr43a-GAL4 in GRNs of the LSO and VCSO ( Fig. 3a,b ). In addition, the brains from poxn null mutants had morphologically normal projections from pharyngeal GRNs, while they lacked the leg projections seen in otherwise wild-type flies ( Fig. 3e,f ). Examining Gr64e-GAL4 expression in the poxn background confirmed these results and additionally demonstrated that labellar taste peg GRNs are also present in poxn mutants ( Fig. 3c,d,g,h ). To ask whether the pharyngeal GRNs of poxn mutants are functional, we expressed GCaMP3 under the control of Gr43a-GAL4 in the poxn null mutant background, and measured calcium responses during ingestion of sweet compounds. We observed robust activation of Gr43a + pharyngeal GRNs on ingestion of fructose and glycerol but not sorbitol ( Fig. 3i ). Due to the technical difficulties in stimulating flies lacking external taste sensation to ingest sweet tastants during calcium imaging, we did not expand our analysis to a larger panel of compounds. However, it is very likely that poxn Gr43a + pharyngeal neurons retain the same receptive fields seen in a wild-type background ( Fig. 2e ). By contrast, Gr64e + taste peg GRNs did not respond to any of the sweet compounds tested but were activated by carbonated water ( Fig. 3j ), as previously reported for taste pegs in a wild-type background [32] . Together, these data demonstrate unequivocally that poxn mutants retain functional pharyngeal taste sensilla that are capable of responding to sweet compounds. Moreover, while functional taste peg GRNs also exist in these mutants, they do not respond to sweet compounds, and thus are unlikely to affect our subsequent behavioural analyses of sweet taste preferences driven by the pharyngeal sense organs. 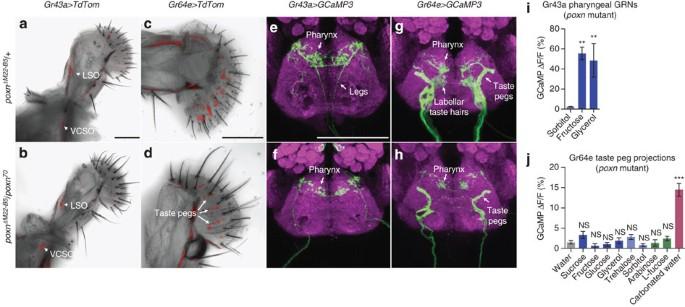Figure 3:poxnnull mutants retain functional pharyngeal sense organs. (a,b) Pharyngeal GRNs labelled byGr43a-GAL4drivingUAS-TdTomatoinpoxnΔM22-B5/+ heterozygotes (a) andpoxnΔM22-B5/poxn70null mutants (b). Arrows point to GRNs in the LSO and VCSO. (c,d) Labellar GRNs labelled byGr64e-GAL4drivingUAS-TdTomatoinpoxnΔM22-B5/+ heterozygotes (a) andpoxnΔM22-B5/poxn70null mutants (b). Arrows point to taste peg GRNs ind. (e–h) Immunofluorescence of anti-GFP (green) and nc82 (magenta) in the brains ofpoxnΔM22-B5/+ heterozygotes (e,g) andpoxnΔM22-B5/poxn70null mutants (f,h) expressing GCaMP3 under control ofGr43a-GAL4(e,f) orGr64e-GAL4(g,h). Arrows point to GRN projections originating from the various body locations. (i,j) Peak fluorescence changes of GCaMP3 inGr43a-GAL4pharyngeal (i) orGr64e-GAL4taste peg (j) axon terminals inpoxnΔM22-B5/poxn70null mutants during ingestion of the indicated compounds. Values represent mean±s.e.m. forn=5 flies, with data collected over at least 2 days. Asterisks indicate significant difference from sorbitol (i) or water (j) by one-way analysis of variance with Bonferroni correction for multiple comparisons: **P<0.01, ***P<0.001; NS, not significant. Scale bars, 100 μm. Figure 3: poxn null mutants retain functional pharyngeal sense organs. ( a , b ) Pharyngeal GRNs labelled by Gr43a-GAL4 driving UAS-TdTomato in poxn ΔM22-B5 /+ heterozygotes ( a ) and poxn ΔM22-B5 / poxn 70 null mutants ( b ). Arrows point to GRNs in the LSO and VCSO. ( c , d ) Labellar GRNs labelled by Gr64e-GAL4 driving UAS-TdTomato in poxn ΔM22-B5 /+ heterozygotes ( a ) and poxn ΔM22-B5 / poxn 70 null mutants ( b ). Arrows point to taste peg GRNs in d . ( e – h ) Immunofluorescence of anti-GFP (green) and nc82 (magenta) in the brains of poxn ΔM22-B5 /+ heterozygotes ( e , g ) and poxn ΔM22-B5 / poxn 70 null mutants ( f , h ) expressing GCaMP3 under control of Gr43a-GAL4 ( e , f ) or Gr64e-GAL4 ( g , h ). Arrows point to GRN projections originating from the various body locations. ( i , j ) Peak fluorescence changes of GCaMP3 in Gr43a-GAL4 pharyngeal ( i ) or Gr64e-GAL4 taste peg ( j ) axon terminals in poxn ΔM22-B5 / poxn 70 null mutants during ingestion of the indicated compounds. Values represent mean±s.e.m. for n =5 flies, with data collected over at least 2 days. Asterisks indicate significant difference from sorbitol ( i ) or water ( j ) by one-way analysis of variance with Bonferroni correction for multiple comparisons: ** P <0.01, *** P <0.001; NS, not significant. Scale bars, 100 μm. Full size image poxn mutants prefer sweet compounds Given that poxn mutants have functional pharyngeal sweet taste, but apparently lack all peripheral sweet taste sensation, we asked whether pharyngeal taste is sufficient to direct consumption of a variety of sweet compounds. First, we verified that poxn null mutants lack peripheral sweet taste responses by performing the PER [7] , [33] , [34] . We used ribose as a negative control stimulus, as it evokes no significant response from L -type taste sensilla on the labellum [4] . However, our observation that ribose elicits a mean PER response of ~20% in control flies suggests that it may stimulate some appetitive taste neurons at a low level ( Fig. 4 ). Alternatively, these responses could be the result of osmotic differences between the ribose solution and water used to water satiate the flies before testing [35] , [36] . Nevertheless, control flies ( w 1118 ) showed robust PER to all sweet compounds tested, responding at frequencies significantly higher than those elicited by ribose ( Fig. 4a,c ). By contrast, PER was entirely abolished in poxn mutants following stimulation of either the labellum or the tarsal segment of the legs ( Fig. 4b,d ). 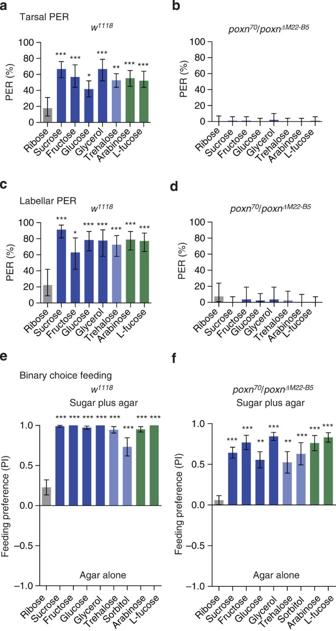Figure 4:poxnnull mutants lack peripheral taste responses but prefer sweet compounds. (a–d) PER responses ofw1118(a,c) andpoxnΔM22-B5/poxn70null mutant (b,d) flies following stimulation of the tarsi (a,b) or labellum (c,d) with the indicated compounds. Values represent percentage of stimulations resulting in a positive response; error bars show 95% binomial confidence interval, and asterisks indicate significant difference from ribose stimulation: *P<0.05, **P<0.01, ***P<0.001 by Fisher’s exact test;n=17–50 flies forw1118tarsal PER,n=17–33 flies forpoxntarsal PER,n=9–19 flies forw1118labellar PER andn=9–17 flies forpoxnlabellar PER. (e,f) Preference ofw1118(e) andpoxnΔM22-B5/poxn70null mutant flies (f) for 100 mM solutions of the indicated compounds in 1% agar versus agar alone. Values represent mean±s.e.m. forn=10 groups of 10 flies each, with independent replicates performed over at least 2 days. Asterisks indicate significant difference from ribose preference by one-way analysis of variance with Bonferroni correction for multiple comparisons: **P<0.01, ***P<0.001. Figure 4: poxn null mutants lack peripheral taste responses but prefer sweet compounds. ( a – d ) PER responses of w 1118 ( a , c ) and poxn ΔM22-B5 / poxn 70 null mutant ( b , d ) flies following stimulation of the tarsi ( a , b ) or labellum ( c , d ) with the indicated compounds. Values represent percentage of stimulations resulting in a positive response; error bars show 95% binomial confidence interval, and asterisks indicate significant difference from ribose stimulation: * P <0.05, ** P <0.01, *** P <0.001 by Fisher’s exact test; n =17–50 flies for w 1118 tarsal PER, n =17–33 flies for poxn tarsal PER, n =9–19 flies for w 1118 labellar PER and n =9–17 flies for poxn labellar PER. ( e , f ) Preference of w 1118 ( e ) and poxn ΔM22-B5 / poxn 70 null mutant flies ( f ) for 100 mM solutions of the indicated compounds in 1% agar versus agar alone. Values represent mean±s.e.m. for n =10 groups of 10 flies each, with independent replicates performed over at least 2 days. Asterisks indicate significant difference from ribose preference by one-way analysis of variance with Bonferroni correction for multiple comparisons: ** P <0.01, *** P <0.001. Full size image Next, we subjected poxn mutants and controls to a variation of the binary feeding choice paradigm in which groups of food-deprived flies were allowed to feed for 2 h on drops of 1% agar with or without a given test compound. Again, we used ribose as a negative control because it has little to no taste response or nutritional value [4] , [26] . Control flies showed a small preference for ribose (preference index (PI)=0.23±0.09) over plain agar, which may be due to weak taste responses or the osmolarity differences discussed above ( Fig. 4e ). This effect was reduced in poxn mutants (PI=0.06±0.06). As expected, poxn mutants and controls displayed robust preference for sucrose, fructose, glucose and glycerol ( Fig. 4f ). All of these compounds are nutritional [23] , [25] , [26] and activate Gr43a + pharyngeal GRNs ( Fig. 2e ). The potential role of nutritional content in guiding feeding decisions is supported by the observation that poxn mutants preferred two compounds, trehalose and sorbitol, that are caloric but did not stimulate pharyngeal GRNs in our experiments ( Fig. 4f ). Importantly, poxn mutants also strongly preferred arabinose and L -fucose, both of which stimulate sugar taste but offer no caloric value [4] , [23] , [25] , [26] . These data strongly suggest that activation of pharyngeal taste neurons is sufficient to drive consumption behaviour, and that this activation accounts for at least part of the previously reported preference of poxn mutants for caloric sugars [21] , [22] . To further examine the role of pharyngeal taste in driving the preference of poxn mutants for sweet compounds, we silenced Gr64e + pharyngeal GRNs in the poxn mutant background through expression of the inward rectifying potassium channel KIR2.1 (ref. 37 ). Importantly, the insertion of Gr64e-GAL4 used ( Gr64e-GAL4 II ) lacks expression in the taste pegs ( Fig. 5a ), meaning that silencing specifically affects pharyngeal GRNs. Silencing of Gr64e + GRN function in poxn mutants resulted in a complete loss of preference for arabinose and L -fucose over agar alone, indicating that Gr64e + pharyngeal GRNs are necessary for the preference for non-caloric sweet sugars in poxn mutants ( Fig. 5b ). This suggests that Gr64e-GAL4 likely labels the complete set of pharyngeal sweet GRNs, and that poxn mutants lacking Gr64e + pharyngeal GRN function may be sweet-blind. 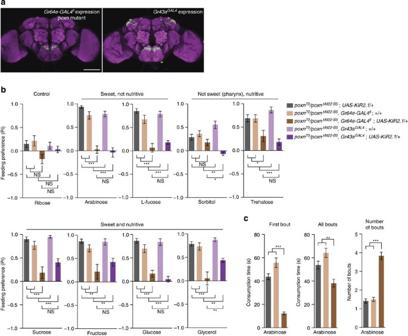Figure 5: Pharyngeal GRNs are necessary for the preference ofpoxnmutants for sweet compounds. (a) Immunofluorescence of anti-GFP (green) and nc82 (magenta), showing expression of theGr64e-GAL4IIandGr43aGAL4drivers used in the behavioural experiments shown.Gr64e-GAL4is shown in apoxnnull mutant background, whileGr43aGAL4is in apoxn/+ heterozygous background. Scale bars, 100 μm. (b) Preference of indicated genotypes for 100 mM solutions of the specified compounds in 1% agar (positive) versus agar alone (negative). (c) Temporal consumption characteristics of the indicated genotypes in response to stimulation with 50 mM arabinose. Values represent mean±s.e.m. forn=10 groups of 10 flies each inbandn=29–60 flies inc, with independent replicates performed over at least 2 days. Asterisks indicate significant difference by one-way analysis of variance with Bonferroni correction for multiple comparisons: *P<0.05, **P<0.01, ***P<0.001; NS, not significant. Figure 5: Pharyngeal GRNs are necessary for the preference of poxn mutants for sweet compounds. ( a ) Immunofluorescence of anti-GFP (green) and nc82 (magenta), showing expression of the Gr64e-GAL4 II and Gr43a GAL4 drivers used in the behavioural experiments shown. Gr64e-GAL4 is shown in a poxn null mutant background, while Gr43a GAL4 is in a poxn /+ heterozygous background. Scale bars, 100 μm. ( b ) Preference of indicated genotypes for 100 mM solutions of the specified compounds in 1% agar (positive) versus agar alone (negative). ( c ) Temporal consumption characteristics of the indicated genotypes in response to stimulation with 50 mM arabinose. Values represent mean±s.e.m. for n =10 groups of 10 flies each in b and n =29–60 flies in c , with independent replicates performed over at least 2 days. Asterisks indicate significant difference by one-way analysis of variance with Bonferroni correction for multiple comparisons: * P <0.05, ** P <0.01, *** P <0.001; NS, not significant. Full size image Since poxn , Gr64e-silenced flies lack both peripheral and identified pharyngeal sweet taste, we used them to re-evaluate the role of post-ingestive nutrient sensing in driving preference for a number of sugars. Silencing of pharyngeal taste caused only a mild, insignificant decrease in the preference of poxn mutant flies for sorbitol ( Fig. 5b ), consistent with previously reported post-ingestive mechanisms promoting consumption of this compound, and its reported tastelessness [13] . However, it is worth noting that the preference for sorbitol in these experiments was weak, so it is difficult to confidently ascribe a taste-independent effect. In contrast to sorbitol, the preference for trehalose was significantly reduced following silencing of Gr64e + pharyngeal GRNs, suggesting that this sugar may stimulate pharyngeal GRNs at a level below the sensitivity of our calcium imaging but enough to affect behaviour. Strikingly, silencing Gr64e + pharyngeal GRNs markedly reduced the preference of poxn flies for all four sweet and nutritive compounds tested ( Fig. 5b ). These data suggest that taste is the dominant driver of feeding preference in our short-term binary choice assay, and, in contrast to previous reports [21] , [22] , taste-independent post-ingestive sugar sensing has little, if any, effect on consumption behaviour in this context. To further probe the factors influencing sugar preference, we repeated the silencing experiment using a GAL4 knock-in allele of Gr43a that is expressed in the same complement of pharyngeal GRNs as Gr64e-GAL4 II but also shows additional expression in identified sugar-sensing neurons in the protocerebrum and a population of neurons in the proventricular ganglion [13] . Consistent with a role for Gr43a + brain neurons in promoting the ingestion of sorbitol, we observed a complete lack of sorbitol preference in Gr43a-silenced poxn mutants ( Fig. 5b ). Notably, this was a significant reduction compared with both genetic controls and Gr64e-silenced flies. Interestingly, while the behavioural assay used may lack the resolution to tease out small differences between Gr64e and Gr43a silencing, we observed a trend towards increased preference for sweet and nutritive sugars in Gr43a-silenced mutants compared with Gr64e-silenced flies. This trend, which was insignificant for sucrose and fructose but significant for glycerol, could reflect weaker silencing with the Gr43a GAL4 driver, a difference in genetic background, or the previously reported role for Gr43a + brain neurons in promoting feeding termination of nutritive sweet sugars in some contexts [13] . Nevertheless, overall, our silencing results strongly support the conclusion that short-term sugar preferences are primarily taste-mediated, even in poxn mutants lacking external gustatory sensilla. Pharyngeal sweet GRNs sustain ingestion On the basis of the anatomical position of pharyngeal GRNs, we wondered whether they might affect food preference by preferentially sustaining the ingestion of sweet compounds. To test this, we subjected poxn , Gr64e-silenced flies to a temporal consumption assay [38] and compared their behaviour with that of the poxn controls with intact pharyngeal GRN function ( Fig. 5c ). We found that poxn flies with silenced pharyngeal GRNs displayed a dramatic reduction in the duration of consumption during the first bout of feeding on a solution of sweet, non-nutritive arabinose compared with non-silenced controls, as well as a reduction in total feeding time over multiple bouts and an elevated number of feeding bouts before ‘satiety’ (defined here as the refusal to initiate further feeding). These data support the notion that pharyngeal GRNs indeed function to sustain ingestion of sweet, appetitive food sources. Much is known about sugar sensing through peripheral sweet taste neurons in the fly’s legs and labellum, and there is growing interest in mechanisms that sense dietary sugars following ingestion [39] , [40] . Sugar sensing by the pharyngeal sense organs, however, has remained virtually unexplored due to their inaccessibility to electrophysiology and the lack of genetic tools to specifically manipulate their function. This represents an important gap in our understanding of how sugar feeding is regulated, since the pharyngeal sense organs must operate following the initiation of feeding, but before ingestion. They are, therefore, poised to provide feedback during feeding, contributing to the ongoing decision of whether to maintain or terminate ingestion. Our calcium imaging data demonstrated that the receptive fields of pharyngeal sweet GRNs are in line with predictions based on the receptor expression and specificities [4] , [5] , [10] , [11] , [13] , [15] , [41] . All putative pharyngeal sweet GRNs co-express Gr43a and Gr64e, which are receptors tuned to fructose and glycerol, respectively, and we observed robust calcium responses to those two compounds. Expression of Gr61a in the LSO likely accounts for the response to glucose, since Gr61a-dependent glucose responses are seen in tarsal GRNs lacking Gr5a [41] . Likewise, sucrose and L -fucose responses can be accounted for by the expression of Gr64a in the LSO [4] , [5] , [10] . Notably, we did not observe responses to trehalose, consistent with the lack of Gr5a expression, which is necessary for trehalose responses in the labellum [4] . However, our behavioural data suggested that Gr64e + pharyngeal GRNs mediate some attraction to trehalose. This apparent discrepancy could be explained if trehalose excites sweet pharyngeal GRNs at a level too low to observe significant calcium responses in our preparation, a possibility supported by previous reports that overexpression of Gr43a or Gr64e confers trehalose sensitivity to tarsal GRNs or ab1C olfactory receptor neurons, respectively [5] , [13] . Using poxn mutants lacking peripheral taste, we demonstrated that pharyngeal sweet GRNs are sufficient to drive preference for sweet compounds in binary choice feeding assays. These results indicate that appetitive taste is not absolutely necessary for feeding initiation, and that flies must ‘sample’ potential food sources in the absence of sweet taste input from the legs and labellum. Moreover, we provide evidence that activation of pharyngeal sweet GRNs prolongs feeding by providing a positive feedback signal to sustain ingestion. This proposed role for pharyngeal GRN function is also consistent with their physiology, which exhibits prolonged activation during consumption of sweet compounds compared with previously reported responses in the labellum [6] , [31] . It is likely that this prolonged activation functions to maintain ingestion during feeding bouts lasting up to several seconds. In the future, it will be interesting to examine whether pharyngeal sweet taste plays any specific roles outside of feeding. For example, pharyngeal bitter GRNs appear to be important in selection of egg laying substrates [42] . A key component of our work is the demonstration that poxn mutants have a functional pharyngeal taste system that is critical in guiding their preference for sweet compounds, which therefore precludes their experimental use as ‘taste-blind’ flies. The behavioural preference we observed of poxn mutant flies for the non-nutritional sweetners L -fucose and arabinose contrasts with the conclusion reached by Dus et al. [21] , who performed a similar experiment with the artificial sweetner sucralose. One possible explanation for this difference is that arabinose and L -fucose may activate pharyngeal sweet GRNs more potently than sucralose. Another possible source of the discrepancy is that Dus et al. [21] analysed their feeding data by plotting the total proportion of flies to eat each option in the binary choice assay, while we analysed relative preference between the options. Nevertheless, the strong dependence of poxn mutants on Gr64e + GRNs for preferred consumption of both nutritive and non-nutritive sweeteners demonstrates that the majority of the preference of these mutants for sweet compounds is mediated by pharyngeal taste sensitivity. By silencing Gr64e + GRNs in a poxn mutant background, we created for the first time a fly that may completely lack sweet taste, allowing one to re-evaluate the taste-independent role for nutrient-sensing mechanisms in behaviour. While we did observe some evidence for taste-independent selection of nutritive carbohydrates, the observed effect was much weaker than previously suggested [21] , [22] . Although ample additional evidence supports the existence of taste-independent carbohydrate sensing [13] , [23] , [24] , [25] , [26] , its specific role in regulating feeding remains unclear. Why do we observe such weak preference of putatively sweet-blind flies for nutritive sugars? One possibility is the particular behavioural assay used, which operates over only 2 h. We have previously reported increasing effects of caloric content on feeding preferences over the course of a 16-h assay [26] . It will be instructive to re-evaluate the feeding behaviour of poxn , sweet GRN-silenced flies over longer time periods using different behavioural paradigms. Our newly established putatively sweet-blind flies also afford the opportunity to examine potential nutrient-sensing mechanisms in a taste-independent context. For example, by comparing Gr43a-silenced with Gr64e-silenced flies in a poxn mutant background, we were able to observe effects for non-taste Gr43a + populations that are largely consistent with those previously reported [13] . Further evaluation of these and other putative nutrient-sensing cell populations in a sweet taste-blind background will continue to shed light on the apparently complex interactions between the taste-dependent and taste-independent mechanisms that ultimately guide critical feeding decisions. Fly stocks Flies were raised on standard cornmeal fly food at 25 °C and 70% relative humidity. The following fly lines were used: Gr5a-GAL4 , Gr43a-GAL4 , Gr64a-GAL4 , Gr61a-GAL4 , Gr64c-GAL4, Gr64d-GAL4 and Gr64e-GAL4 (ref. 16 ); Gr64f LexA and Gr43a GAL4 (ref. 13 ); UAS-GCaMP3 (ref. 43 ); UAS-KIR2.1 (ref. 37 ); UAS-TdTomato and UAS-GFP (Bloomington stock centre); poxn ΔM22-B5 (ref. 44 ); and poxn 70 (ref. 28 ). Immunohistochemistry Immunohistochemistry was carried out as previously described [33] . The primary antibodies used were rabbit anti-GFP (1:1,000, Invitrogen) and mouse nc82 (1:50, DSHB). The secondary antibodies used were goat anti-rabbit Alexa-488 and goat anti-mouse Alexa-568 (Invitrogen). Images are maximum intensity projections of confocal z-stacks acquired using a Leica SP5 II confocal microscope with 25 × water immersion objective. Gr expression mapping Expression of sweet Gr promoter-GAL4 lines was mapped in the three pharyngeal sense organs by visualizing UAS-mCD8::GFP fluorescence in live tissue. Proboscis tissue was dissected and mounted in 80% glycerol in 1 × PBS before imaging with a Leica SP5 laser scanning confocal microscope. For double-driver analysis, the UAS-mCD8::GFP transgene was under the control of two different Gr promoter-Gal4 transgenes and the number of GFP-labelled neurons were compared with those in flies containing a single-Gal4 driver alone. GCaMP imaging Female flies aged 2–12 days were used for calcium imaging. To prepare flies for imaging, they were briefly anaesthetized and all the legs were removed to allow unobstructed access to the proboscis. Using a custom chamber, each fly was mounted by inserting the cervix into individual collars. To further immobilize the head, nail polish was applied in a thin layer to seal the head to the chamber. Melted wax was applied using a modified dental waxer to adhere the fully extended proboscis to the chamber rim. The antennae and associated cuticle covering the SEZ were removed and adult hemolymph-like buffer with ribose [45] was immediately injected into the preparation to cover the exposed brain. A coverslip was inserted into the chamber to keep the proboscis dry and separated from the bath solution. GCaMP3 fluorescence was viewed with a Leica SP5 II laser scanning confocal microscope equipped with a tandem scanner and HyD detector. The relevant area of the SEZ was visualized using the 25 × water objective with an electronic zoom of eight. Images were acquired at a speed of 8,000 lines per second with a line average of four, resulting in collection time of 60 ms per frame at a resolution of 512 × 200 pixels. The pinhole was opened to 2.68 AU. Stimuli were applied to the proboscis using a pulled glass pipette, and flies were allowed to ingest solutions during imaging. The maximum change in fluorescence (Δ F / F ) was calculated as the peak intensity change divided by the average intensity over 10 frames before stimulation. Behavioural assays For PER, adult female flies were aged 3–10 days and starved on 1% agar at room temperature (~22 °C) for 24 h before testing. For tarsal PER, flies were mounted on glass slides using nail polish. For labellar PER, flies were placed inside a pipette tip cut to size so that only the head was exposed. Flies were then sealed into the tube with tape, and then adhered to a glass slide with double-sided tape. Flies were allowed 1–2 h to recover before testing began. Flies were stimulated with water on their front tarsi or labella for tarsal and labellar PER, respectively, and allowed to drink until satiated. Each fly was then stimulated with a tastant on either the tarsi or labella, and responses to each of three trials were recorded. Flies were provided with water between each tastant. All stimuli were delivered with a 1 ml syringe attached to a 20 μl pipette tip. For statistical purposes, each trial was treated as an independent unit of analysis. Binary choice preference tests were performed similarly to previous descriptions [16] , [21] , [46] . Female flies aged 3–8 days were sorted into groups of 10 at least 2 days before the experiment, and starved on 1% agar at room temperature (~22 °C) for 24 h before testing. For the assay, flies were transferred into standard vials containing six 10 μl dots of agar that alternated in colour. The agar substrates were 1% agar with or without the test stimulus at a concentration of 100 mM. Each choice contained either 0.125 mg ml −1 blue (Erioglaucine, FD&C Blue#1) or 0.5 mg ml −1 red (Amaranth, FD&C Red#2) dye, and half the replicates for each stimulus were done with the dyes swapped to control for any dye preference. Flies were allowed to feed for 2 h in the dark at 25 °C and then frozen and scored for abdomen colour. PI for sugar was calculated as ((number of flies labelled with the stimulus colour)−(number of flies labelled with the plain agar colour))/(total number of flies that fed). The temporal consumption assay was performed on flies deprived of food for 24 h (ref. 38 ). As described above for PER, flies were mounted on glass slides using nail polish and allowed to recover for 1–2 h in a humidified chamber. Water-satiated flies were then offered 50 mM arabinose on their labella. Once they initiated feeding, the time between starting and stopping their first feeding bout was recorded (first bout length). The fly was then offered arabinose again and if they failed to reinitiate feeding for three consecutive stimulations, the assay was terminated for that fly. If flies began a new bout of feeding on stimulation, the time of the subsequent bouts was added to the first bout to determine total consumption time and the number of bouts was recorded. Statistical analyses For PER analyses, the 95% binomial confidence interval was calculated using JavaStat ( http://statpages.org/confint.html ). Fisher’s exact tests were calculated using Graphpad QuickCalcs ( http://www.graphpad.com/quickcalcs/ ). All other statistical tests were performed using GraphPad Prism 6 or SPSS software. No statistical test was used to predetermine sample size. Sample size ranges were chosen based on previously published examples of the same assays. How to cite this article: LeDue, E. E. et al. Pharyngeal sense organs drive robust sugar consumption in Drosophila . Nat. Commun. 6:6667 doi: 10.1038/ncomms7667 (2015).